Breast cancer cells condition lymphatic endothelial cells within pre-metastatic niches to promote metastasis Breast cancer metastasis involves lymphatic dissemination in addition to hematogenous spreading. Although stromal lymphatic vessels (LVs) serve as initial metastatic routes, roles of organ-residing LVs are underinvestigated. Here we show that lymphatic endothelial cells (LECs), a component of LVs within pre-metastatic niches, are conditioned by triple-negative breast cancer (TNBC) cells to accelerate metastasis. LECs within the lungs and lymph nodes, conditioned by tumour-secreted factors, express CCL5 that is not expressed either in normal LECs or in cancer cells, and direct tumour dissemination into these tissues. Moreover, tumour-conditioned LECs promote angiogenesis in these organs, allowing tumour extravasation and colonization. Mechanistically, tumour cell-secreted IL6 causes Stat3 phosphorylation in LECs. This pStat3 induces HIF-1α and VEGF, and a pStat3-pc-Jun-pATF-2 ternary complex induces CCL5 expression in LECs. This study demonstrates anti-metastatic activities of multiple repurposed drugs, blocking a self-reinforcing paracrine loop between breast cancer cells and LECs. The lymphatic endothelium (LE), which comprises lymphatic endothelial cells (LECs), is a specialized endothelium and is distinct from the vascular endothelium. It lacks erythrocytes in the lumen and a well-defined basement membrane [1] . Due to the leaky nature of the LE, lymphatic vessels (LVs) function as a reservoir for the lymph fluid consisting of proteins and cells that have leaked from the vascular system, and transport it back from the tissues to the circulatory system. In cancer, however, the prevailing view is that LVs are routes for cancer metastasis [2] . Numerous studies have shown that tumour LVs serve as initial routes for metastasis. However, mechanisms of lymphogenous metastasis and, particularly, roles of organ-residing LVs in metastasis are not well understood, despite the broad distribution of the LVs throughout the body. Gene expression in LECs is distinct from those in blood endothelial cells (BECs) [3] , [4] , thus LV-mediated metastasis could be modulated by LEC-derived factors. For example, it is known that stromal LECs attract tumour cells into the LVs by expressing CXCL12 and CCL21, chemokine ligands of CXCR4 and CCR7; CXCR4 and CCR7 are chemokine receptors expressed in several types of cancer cells [5] , [6] . We asked what other LEC-derived factors, including chemokines, angiogenesis factors or cytokines, play a role in breast cancer metastasis, since we have observed that secretion profiles of LECs are diverse and abundant, comparable to those of MDA-MB-231 (referred to below as MB231 for brevity) breast cancer cells in reverse western assays for 55 angiogenesis-related factors and 31 chemokines ( Supplementary Fig. 1 ). We previously showed that treatment of animals with tumour-conditioned media (TCM) prepared from triple-negative breast cancer (TNBC) cells accelerates lung and lymph node (LN) metastasis [7] . We employed two different subtypes of TNBC cell lines: mesenchymal-like MDA-MB-231 and basal-like SUM149 (ref. 8 ). In that study, we observed that the lungs and LNs from TCM-treated animals had 2–4 times elevation in organ-residing LECs, implying increased lymphangiogenesis, compared with serum-free media (SFM)-treated animals. Strikingly, the TCM-treated group also showed 3–10 times more metastases in those organs within 4 weeks in the MDA-MB-231 model and 6 weeks in the SUM149 model, which is significantly faster than SFM-treated animals as well as current spontaneous metastasis models that take more than 7–10 weeks [9] . This unexpected increase in metastasis led us to hypothesize that there are unknown signalling pathways among three partners: tumour-secreted factors (TCM), organ-residing LECs and tumour cells. In this study, we investigate how TCM-induced organ-residing LECs influence metastasis and propose novel mechanisms of metastasis as well as possible targets for therapeutic intervention for metastatic breast cancer. Here we employ a ‘tumour-conditioned LEC’ model, which involves TCM-treated LECs in vitro or in vivo ; this simulates the pro-metastatic effects of tumour-secreted factors in advanced breast cancer patients. In this report, we document for the first time that LECs within pre-metastatic organs are conditioned by tumour-secreted factors, and start to express CCL5 and vascular endothelial growth factor (VEGF), facilitating tumour cell recruitment, extravasation and colonization. We show that interleukin 6 (IL6) secreted by the tumour cells activates Stat3 pathways in LECs, resulting in lymphatic expression of CCL5 and VEGF. We propose central players for TNBC metastasis and test diverse repurposed drug agents to inhibit metastatic disease. Tumour-conditioned LECs express CCL5 Tumour-conditioned LECs (MB231-LECs) were prepared by growing normal LECs (n-LECs) in 30% TCM (TCM:EGM=3:7; EGM, endothelial growth media). We discovered that expression of CCL5 and CXCL7 was highly increased in MB231-LECs, compared with n-LECs ( Fig. 1a ). Since CXCL7 was also expressed in MB231 cells ( Supplementary Fig. 2a ), we focused on CCL5. CCL5 expression in MB231-LECs plateaued at day 2 ( Fig. 1b ), showing very high expression of CCL5 compared with n-LECs and MB231 cells ( Fig. 1c ). Another TNBC cell line, SUM149, and an oestrogen receptor-positive (ER+) breast cancer cell line, MCF7, were also tested: SUM149-TCM promoted CCL5 expression in LECs, however, MCF7-TCM did not ( Fig. 1d ). 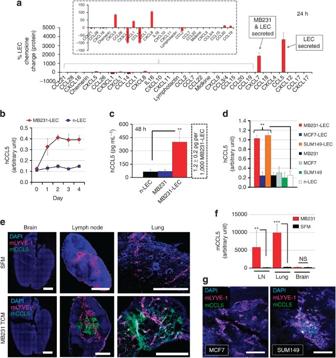Figure 1: Tumour-conditioned LECs (MB231-LECs) express CCL5. (a) Reverse western assays with the human chemokine antibody arrays (R&D Systems) detected the relative level of 31 chemokines expressed in n-LECs or tumour-conditioned LECs (MB231-LECs). MB231-LECs were prepared by growing n-LECs in 30% TCM media for 4 days. The media were replaced with 3 ml SFM with 2% FBS. After 48 h, the supernatant was centrifuged and filtered. The resulting MB231-LEC-CM (MB231-LEC-CM) were analysed, comparing with n-LEC-CM. (b) ELISAs for human CCL5 (Quantikine ELISA, R&D System) performed on MB231-LEC and n-LEC-CM. MB231-LEC-CM and n-LEC-CM were obtained at days 0, 1, 2, 3 and 4 of TCM induction, and we showed accumulation of CCL5 plateauing at day 2 (n=4). (c) CCL5 concentration in each CM was determined at 48 h by CCL5 ELISAs. CCL5 expression in MB231-LECs was significantly higher than that in n-LECs (**P=0.0023) or in MB231 (**P=0.0038). MB231-LECs (1,000) expressed 1.2±0.2 pg hCCL5 in 48 h (n=3). (d) LEC was treated with TCM obtained from MCF7, MB231 and SUM149 cells. MB231- and SUM149-TCM induced CCL5 expression in LECs, compared with the secretion from n-LECs (**P<0.01); however, MCF7-TCM were inactive (n=3). (e) TCM (50 μl) prepared from MB231, SUM149 and MCF7 cells or SFM were subcutaneously administered into nude mice (4–5 weeks, female, NCI) for 2 weeks. Excised organs (brains, Br-LNs, lungs) were fixed, frozen, sectioned and probed with anti-mouse LYVE-1 and anti-mouse CCL5 antibodies. LNs and lungs from MB231-TCM-treated animals showed mCCL5 expression around mLVs. No mCCL5 expression was seen in the LNs and lungs from the SFM-treated groups, and the brains from either group. LVs are absent in the brains. Scale bar, 1 mm. (f) mCCL5 pixel density was quantified by ImageJ (**P=0.0048, ***P=0.00075,n=12). (g) MCF7-TCM or SUM149-TCM was injected into the animals for two weeks after which lungs were collected, fixed, sectioned and probed with anti-mouse LYVE-1 and anti-mouse CCL5 antibodies. SUM149-TCM treatment induced mCCL5 expression in lungs, while MCF7-TCM treatment did not. Figure 1: Tumour-conditioned LECs (MB231-LECs) express CCL5. ( a ) Reverse western assays with the human chemokine antibody arrays (R&D Systems) detected the relative level of 31 chemokines expressed in n-LECs or tumour-conditioned LECs (MB231-LECs). MB231-LECs were prepared by growing n-LECs in 30% TCM media for 4 days. The media were replaced with 3 ml SFM with 2% FBS. After 48 h, the supernatant was centrifuged and filtered. The resulting MB231-LEC-CM (MB231-LEC-CM) were analysed, comparing with n-LEC-CM. ( b ) ELISAs for human CCL5 (Quantikine ELISA, R&D System) performed on MB231-LEC and n-LEC-CM. MB231-LEC-CM and n-LEC-CM were obtained at days 0, 1, 2, 3 and 4 of TCM induction, and we showed accumulation of CCL5 plateauing at day 2 ( n =4). ( c ) CCL5 concentration in each CM was determined at 48 h by CCL5 ELISAs. CCL5 expression in MB231-LECs was significantly higher than that in n-LECs (** P =0.0023) or in MB231 (** P =0.0038). MB231-LECs (1,000) expressed 1.2±0.2 pg hCCL5 in 48 h ( n =3). ( d ) LEC was treated with TCM obtained from MCF7, MB231 and SUM149 cells. MB231- and SUM149-TCM induced CCL5 expression in LECs, compared with the secretion from n-LECs (** P <0.01); however, MCF7-TCM were inactive ( n =3). ( e ) TCM (50 μl) prepared from MB231, SUM149 and MCF7 cells or SFM were subcutaneously administered into nude mice (4–5 weeks, female, NCI) for 2 weeks. Excised organs (brains, Br-LNs, lungs) were fixed, frozen, sectioned and probed with anti-mouse LYVE-1 and anti-mouse CCL5 antibodies. LNs and lungs from MB231-TCM-treated animals showed mCCL5 expression around mLVs. No mCCL5 expression was seen in the LNs and lungs from the SFM-treated groups, and the brains from either group. LVs are absent in the brains. Scale bar, 1 mm. ( f ) mCCL5 pixel density was quantified by ImageJ (** P =0.0048, *** P =0.00075, n =12). ( g ) MCF7-TCM or SUM149-TCM was injected into the animals for two weeks after which lungs were collected, fixed, sectioned and probed with anti-mouse LYVE-1 and anti-mouse CCL5 antibodies. SUM149-TCM treatment induced mCCL5 expression in lungs, while MCF7-TCM treatment did not. Full size image We next checked for TCM-induced CCL5 expression in vivo , employing athymic nude mice (female, 5 weeks, NCI) to minimize the effect of T lymphocytes on CCL5 expression. CCL5 is also known as RANTES (regulated upon activation, normal T cell expressed and secreted), since T lymphocytes express and secrete it [10] . We injected 50 μl of SFM or TCM prepared from MB231, SUM149 or MCF7 breast cancer cells subcutaneously as previously described [7] , [11] . Mouse LVs (mLVs) in the LNs and lungs from the animals treated with MB231- or SUM149-TCM expressed mouse CCL5 (mCCL5), whereas the mLVs in animals treated with MCF7-TCM or SFM did not ( Fig. 1e–g ). Brain tissues where LVs are absent did not show mCCL5 expression on MB231-TCM treatment ( Fig. 1e,f ). We assessed the concentration of mCCL5 in TCM-treated animals ( Supplementary Fig. 3 ). We did not inoculate tumour cells in these animals so that we could measure mCCL5 that was induced only by the TCM ( Supplementary Fig. 3a ). TCM treatment induced mCCL5 in these animals; more than 450 pg ml −1 mCCL5 was present in the mouse plasma ( Supplementary Fig. 3b ). TCM-induced mCCL5 was not associated with alpha smooth muscle actin (αSMA), a marker of myofibroblasts or pericytes ( Supplementary Fig. 2b ). Possible association of mCCL5 with mouse CD45 (mCD45)-positive leukocytes, mF4/80-positive macrophages and mIba-1-positive-activated macrophages was also examined ( Supplementary Figs 4–6 ). Leukocytes were ubiquitously detected in the lungs in both TCM- and SFM-treated animals ( Supplementary Fig. 4a,b ). Among those leukocytes, Iba-1- or F4/80-positive macrophages were detected in TCM-treated lungs and LNs ( Supplementary Figs 4 and 5 ). Importantly, TCM-induced mCCL5 was not colocalized with the leukocytes and macrophages but was associated with LYVE-1-positive LECs ( Supplementary Fig. 6 ). CCL5 expressed by MB231-LECs drives metastasis We observed that CM obtained from MB231-LECs promotes MB231 cell migration ( Supplementary Fig. 7a ). CCL5 can interact with CCR1/3/5 (ref. 12 ), so we blocked CCR1 by BX513, CCR3 by SB328437 and CCR5 by maraviroc to determine which of these receptors induces MB231 cell migration. Only maraviroc blocked MB231 cell migration ( Fig. 2a,b ). We confirmed that both MB231 and MDA-MB-231-luc-D3H2LN express CCR5 ( Fig. 2c ), suggesting that LEC-secreted CCL5 triggers chemotaxis of MB231 cells. The effect of the CCR5 inhibitor was compared with that of anti-CCR7-neutralizing antibodies in MB231 cell migration assays ( Supplementary Fig. 7b,c ), because CCL21, a chemokine ligand for CCR7, is known as another inducer of lymphatic metastasis [5] . Maraviroc blocked MB231 cell migration induced by MB231-LEC-CM, whereas the anti-CCR7 antibody blocked n-LEC-CM-induced migration, demonstrating that the CCL5-CCR5 axis is essential for tumour cell migration towards tumour-conditioned LECs rather than towards physiological LECs. 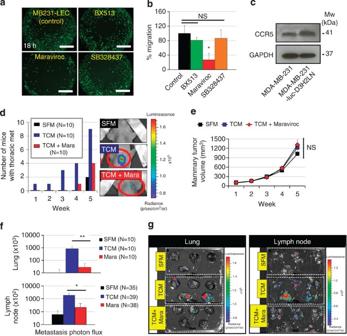Figure 2: MB231-LECs promote metastasis through the CCL5-CCR5 axis. (a) MB231 cells were pre-labelled with Cell Tracker Green and their migration was assessed using the Oris cell migration kit. Labelled MB231 cells (50,000) in complete media were added to each well of a 96-well plate containing stoppers to prevent the cells from settling in the centre region of the wells. Cells were allowed to adhere for 4 h, after which the stoppers were carefully removed. MB231-LEC-CM with or without inhibitors were added, and the cells that migrated to the centre of the well were quantified by measuring the fluorescence at 485/530 nm (n=4). Maraviroc, a CCR5 inhibitor, potently blocked MB231 cell migration in the presence of MB231-LEC-CM at 18 h. Scale bar, 500 μm. (b) Fluorescent signal from the migrated cells fromawas measured at 485/530 nm and quantified (*P=0.013,n=4). (c) Human CCR5 levels in 300,000 MB231 and luc-MB231 cells were measured by western blotting. GAPDH was used as a loading control. (d) Athymic nude mice (4–5 weeks, female, NCI,n=10) were pretreated with TCM or SFM (50 μl) for 2 weeks before inoculation with luc-MB231 tumour cells and initiation of maraviroc (8 mg kg−1per day, p.o.) or vehicle treatment. Five weeks later, the maraviroc-treated group showed ~50% inhibition of metastasis, compared with vehicle-treated group. Red circles represent thoracic metastasis observed with the IVIS imager. (e) Tumour volume was measured using a caliper (n=10), and the volume was calculated using the formula:V=0.52 × (length) × (width)2. (f) Quantification ofg, luciferase-mediated photon flux from the lungs (n=10) and the LNs (n=35–39) were obtained by using Living Image 3D Analysis (Xenogen; **P=0.008, *P=0.042). (g) Representative organ images under the IVIS imager. Data (b,e,f) are reported as mean±s.e.m. Original gel images of data (c) are presented inSupplementary Fig. 25. NS, nonsignificant. Figure 2: MB231-LECs promote metastasis through the CCL5-CCR5 axis. ( a ) MB231 cells were pre-labelled with Cell Tracker Green and their migration was assessed using the Oris cell migration kit. Labelled MB231 cells (50,000) in complete media were added to each well of a 96-well plate containing stoppers to prevent the cells from settling in the centre region of the wells. Cells were allowed to adhere for 4 h, after which the stoppers were carefully removed. MB231-LEC-CM with or without inhibitors were added, and the cells that migrated to the centre of the well were quantified by measuring the fluorescence at 485/530 nm ( n =4). Maraviroc, a CCR5 inhibitor, potently blocked MB231 cell migration in the presence of MB231-LEC-CM at 18 h. Scale bar, 500 μm. ( b ) Fluorescent signal from the migrated cells from a was measured at 485/530 nm and quantified (* P =0.013, n =4). ( c ) Human CCR5 levels in 300,000 MB231 and luc-MB231 cells were measured by western blotting. GAPDH was used as a loading control. ( d ) Athymic nude mice (4–5 weeks, female, NCI, n =10) were pretreated with TCM or SFM (50 μl) for 2 weeks before inoculation with luc-MB231 tumour cells and initiation of maraviroc (8 mg kg −1 per day, p.o.) or vehicle treatment. Five weeks later, the maraviroc-treated group showed ~50% inhibition of metastasis, compared with vehicle-treated group. Red circles represent thoracic metastasis observed with the IVIS imager. ( e ) Tumour volume was measured using a caliper ( n =10), and the volume was calculated using the formula: V =0.52 × (length) × (width) 2 . ( f ) Quantification of g , luciferase-mediated photon flux from the lungs ( n =10) and the LNs ( n =35–39) were obtained by using Living Image 3D Analysis (Xenogen; ** P =0.008, * P =0.042). ( g ) Representative organ images under the IVIS imager. Data ( b , e , f ) are reported as mean±s.e.m. Original gel images of data ( c ) are presented in Supplementary Fig. 25 . NS, nonsignificant. Full size image We next pretreated animals with TCM or SFM daily for 2 weeks, followed by inoculation of 2 × 10 6 MDA-MB-231-luc-D3H2LN breast cancer cells into the upper inguinal mammary fat pads and treatment with maraviroc (8 mg kg −1 per day, per os (p.o.)) or vehicle ( Supplementary Fig. 8a ). At week 5, 9 out of 10 mice in the TCM-treated group had metastases, while only 2 out of 10 mice in the SFM-treated group had them. In the maraviroc-treated group, only four mice had metastases showing the anti-metastatic effect of maraviroc ( Fig. 2d ). Primary tumour growth was not influenced by the treatment ( Fig. 2e ). Maraviroc treatment inhibited metastasis in the lungs and LNs, as shown by the reduced photon flux in the organs ( Fig. 2f,g ). The hearts, brains, spleens and livers did not show significant metastases ( Supplementary Fig. 8b,c ). Next, the effect of maraviroc was assessed in spontaneous metastasis models without TCM pretreatment. We showed potent prevention of lung and LN metastasis by maraviroc treatment in these models as well ( Supplementary Fig. 9 ). These results demonstrate that the CCL5-CCR5 axis is pivotal for lung and LN metastasis in TCM-induced and spontaneous metastasis models and that it can be targeted to inhibit metastasis. MB231-LECs have abnormal expression of angiogenesis factors We discovered that subcutaneous matrigel (500 μl per injection) mixed with LECs (2 × 10 6 ) induced moderate intra-gel angiogenesis in vivo ( Supplementary Fig. 10a ). We screened for angiogenesis-related factors in LEC-CM, using a reverse western array spotted with antibodies for 55 angiogenesis-related factors ( Supplementary Fig. 10b ). LEC-secreted pro-angiogenic factors (angiogenin, endothelin, HB-EGF, IGFBP-2, MMP-9, PDGF-AA, PlGF), inflammatory factors (CD26, IL-1β, IL-8, CCL2) and anti-angiogenic factors (angiopoietin-2, endostatin, pentraxin-3, serpin-E1, TIMP-1, IGFBP-3) into the CM (LEC-CM; Supplementary Fig. 10c ). Although LEC-CM moderately induced EC proliferation, the rate of proliferation was far smaller than that in EGM-2, suggesting that LEC-secreted anti- and pro-angiogenic factors are in balance for angiogenic homeostasis or that LEC-secreted pro-angiogenic factors are not sufficient to trigger angiogenesis ( Supplementary Fig. 10d,e ). We hypothesized that the angiogenic homeostasis in LECs can be perturbed by TCM treatment. To address this question in vivo , matrigels mixed with LECs (LEC-matrigel group) were implanted into animals followed by systemic subcutaneous administration of TCM or SFM for 2 weeks ( Fig. 3 ). For controls, ‘HUVEC-matrigel’ and ‘no cell’ groups were prepared. Strikingly, profound intra-gel angiogenesis was observed in the TCM-treated LEC-matrigel group ( Fig. 3a ). ‘HUVEC group’ or ‘no cell group’ showed relatively less angiogenesis. Tail-vein injection of fluorescein isothiocyanate (FITC)-dextran (70 kDa) visualized angiogenesis in the plugs ( Fig. 3b,c ). Infiltration of the host blood vessels (BVs) into the plugs was also observed ( Fig. 3d ). Immunostaining with anti-mCD31 ( Fig. 3e,f ) and anti-lectin antibodies ( Supplementary Fig. 11 ) showed that the recruitment of the host BVs was increased by TCM. Anti-hVEGFR3 staining was performed to detect human LECs previously included in the matrigel plugs ( Fig. 3e,f ). 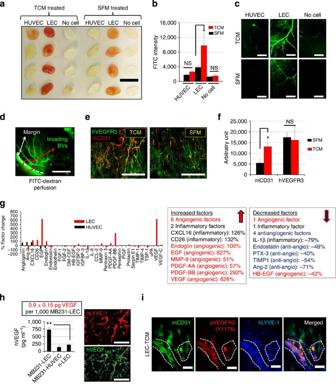Figure 3: MB231-LECs promote angiogenesisin vivo. (a) Matrigel plug assays with LECs/HUVECs or without cells. Matrigel (500 μl) containing LECs or HUVECs (2 × 106per gel) and heparin (10 U per gel) was injected subcutaneously on the ventral side of both flanks of nude mice. TCM or SFM (50 μl) were subcutaneously administered daily for 10 days, the mice were killed and the gel plugs were excised and analysed. Scale bar, 10 mm. (b) One hour before killing, FITC-dextran (70 kDa) was injected through the tail vein to visualize BVs in the gel plugs. Plugs were homogenized and the intensity of FITC was measured and normalized to the volume of the plug (*P=0.030,n=4). (c) Representative FITC images of the gel plugs under the fluorescent microscope. Scale bar, 200 μm. (d) A representative image showing the margin of the plugs. Mouse BVs (mBVs) infiltrate the plug. Scale bar, 500 μm. (e) Gel plugs were fixed, frozen, sectioned and stained with anti-hVEGFR3 (green) and anti-mCD31 (red) antibodies to detect hLECs and mBVs. Scale bar, 500 μm. (f) Quantification ofe. (*P=0.037,n=12). (g) Reverse western assays with human angiogenesis antibody arrays detected the relative changes of 55 angiogenesis factors in LECs and HUVECs after tumour conditioning. Profiles of LEC-derived factors (enhanced or downregulated) are described in the box (the right panel). TCM did not induce any significant changes in HUVECs (n=2). (h) hVEGF concentration (pg ml−1) in each CM was determined by ELISAs (**P=0.0084,n=3). MB231-LECs (1,000) secreted 0.9±0.15 pg of VEGF. Immunostaining of LEC-matrigel plugs revealed that hVEGF165(green) expression was colocalized with hLECs (hLYVE-1, red). Scale bar, 200 μm (right panel). (i) LEC-matrigel from TCM-treated animals showed phospho-VEGFR2 (Y1175, red) around areas that were positive for mCD31 (green) and hLYVE-1 (blue) signals. Scale bar, 100 μm. Data (b,f,g,h) are reported as mean±s.e.m. NS, nonsignificant. Figure 3: MB231-LECs promote angiogenesis in vivo . ( a ) Matrigel plug assays with LECs/HUVECs or without cells. Matrigel (500 μl) containing LECs or HUVECs (2 × 10 6 per gel) and heparin (10 U per gel) was injected subcutaneously on the ventral side of both flanks of nude mice. TCM or SFM (50 μl) were subcutaneously administered daily for 10 days, the mice were killed and the gel plugs were excised and analysed. Scale bar, 10 mm. ( b ) One hour before killing, FITC-dextran (70 kDa) was injected through the tail vein to visualize BVs in the gel plugs. Plugs were homogenized and the intensity of FITC was measured and normalized to the volume of the plug (* P =0.030, n =4). ( c ) Representative FITC images of the gel plugs under the fluorescent microscope. Scale bar, 200 μm. ( d ) A representative image showing the margin of the plugs. Mouse BVs (mBVs) infiltrate the plug. Scale bar, 500 μm. ( e ) Gel plugs were fixed, frozen, sectioned and stained with anti-hVEGFR3 (green) and anti-mCD31 (red) antibodies to detect hLECs and mBVs. Scale bar, 500 μm. ( f ) Quantification of e . (* P =0.037, n =12). ( g ) Reverse western assays with human angiogenesis antibody arrays detected the relative changes of 55 angiogenesis factors in LECs and HUVECs after tumour conditioning. Profiles of LEC-derived factors (enhanced or downregulated) are described in the box (the right panel). TCM did not induce any significant changes in HUVECs ( n =2). ( h ) hVEGF concentration (pg ml −1 ) in each CM was determined by ELISAs (** P =0.0084, n =3). MB231-LECs (1,000) secreted 0.9±0.15 pg of VEGF. Immunostaining of LEC-matrigel plugs revealed that hVEGF 165 (green) expression was colocalized with hLECs (hLYVE-1, red). Scale bar, 200 μm (right panel). ( i ) LEC-matrigel from TCM-treated animals showed phospho-VEGFR2 (Y1175, red) around areas that were positive for mCD31 (green) and hLYVE-1 (blue) signals. Scale bar, 100 μm. Data ( b , f , g , h ) are reported as mean±s.e.m. NS, nonsignificant. Full size image To understand these in vivo results, angiogenesis factors expressed in LECs/human umbilical vein endothelial cells (HUVECs) after TCM treatment were assessed and compared with n-LEC/HUVEC secretomes ( Fig. 3g ). LEC-derived angiogenic factors that increased after TCM treatment were Endoglin, EGF, MMP-9, PDGF-AA, PDGF-BB and VEGF. At the same time, four anti-angiogenic factors, including endostatin, pentraxin-3 (PTX-3), TIMP-1, and angiopoietin-2 were decreased ( Fig. 3g ). The factors secreted by HUVECs did not change after TCM treatment. VEGF was dramatically increased in MB231-LEC-CM as seen by enzyme-linked immunosorbent assays (ELISAs) ( Fig. 3h , left). Immunostaining of TCM-treated LEC-matrigel plugs also showed that hVEGF 165 is colocalized with hLYVE-1-positive human LECs ( Fig. 3h , right). Phospho-VEGFR2 (Y1175) was detected around hLECs and mBVs, showing that the LEC-secreted hVEGF 165 could activate VEGFR2 signalling pathways ( Fig. 3i ). Although EGF was highly expressed in MB231-LECs ( Fig. 3g ), its angiogenic activity was not significant ( Supplementary Fig. 12 ). MB231-LECs show angiogenic phenotypes EC proliferation, migration, adhesion and tube formation were assessed in MB231-LEC-CM ( Fig. 4a,b ). MB231-LEC-CM promoted HUVEC proliferation, migration and adhesion, compared with n-LEC-CM ( Fig. 4a ). Although robust HUVEC tube formation was observed in MB231-LEC-CM, LEC tube formation was relatively poor in the same CM ( Fig. 4b ), suggesting that the MB231-LEC-CM primarily promotes angiogenesis rather than lymphangiogenesis, which is consistent with very low VEGF-C expression in MB231-LECs ( Fig. 3g ). We next generated growth factor-depleted TCM (GF-dep-TCM) by using anti-hVEGF 165 - and anti-hEGF-neutralizing antibodies ( Supplementary Fig. 13a ). HUVEC adhesion assays confirmed that the immunodepletion was successful ( Supplementary Fig. 13b ). The immunodepletion was performed because both the TCM containing hVEGF 165 and hEGF and the TCM-induced mVEGF 164 in the mouse can promote angiogenesis in vivo , thus complicating interpretation of angiogenesis effects. The use of the GF-dep-TCM clarifies that ‘TCM-induced angiogenesis in vivo ’ is caused by host-derived mVEGF 164 rather than by hVEGF 165 or hEGF already present in TCM ( Supplementary Fig. 14a ). 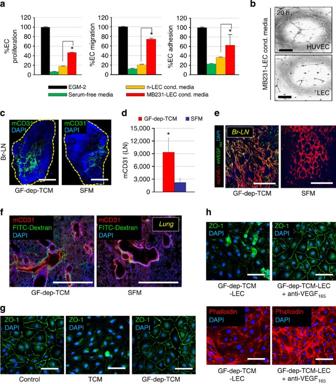Figure 4: GF-dep-TCM promote LN angiogenesis and enhance lung vascular permeability. (a) In the proliferation assays, 2,000 HUVECs per well were plated in 96-well plates and allowed to adhere overnight. On the following day, the media were exchanged with LEC-CM (cond. media), EGM or SFM. Three days later, proliferating cells were quantified at 450 nm by using the WST-1 reagent (*P=0.039,n=6). In the migration assays, 180 μl of EGM-2 or SFM or MB231-LEC-CM were added to the bottom chambers (CIM-plates), HUVECs (45,000 cells per well) were added to the top chamber. The bottom and top chambers were combined, loaded in the RTCA system and the cell index was measured continuously at 20 h (*P=0.011,n=2). In adhesion assays, HUVECs (25,000 cells per well) in 100 μl of EGM-2 or SFM or MB231-LEC-CM were added in E-plates, after which the plate was loaded into the RTCA system. Cell indices at 3 h were analysed (*P=0.042 at 3 h,n=2). (b) HUVEC and LEC tube formation (at 20 h) was induced by MB231-LEC-CM in matrigel matrix. Scale bar, 200 μm. (c) Human growth factor (hVEGF165/hEGF)-depleted TCM (GF-dep-TCM) or SFM were subcutaneously administered daily for 10 days, the nude mice were killed and brachial LNs (Br-LNs) were excised and analysed with anti-mouse CD31 antibodies (green). Scale bar, 1 mm. (d) Quantification ofc(*P=0.032,n=12). (e) Br-LNs from GF-dep-TCM-treated animals were probed with anti-mVEGF164(green); mLV (red). Scale bar, 500 μm. (f) GF-dep-TCM-treated animals were perfused with FITC-dextran (70 kDa) 1 h before termination. Collected lungs were stained with anti-mCD31 (red); dextran (green). Scale bar, 1,000 μm. (g) Anti-ZO-1 antibody staining (green) of HUVEC monolayers treated with SFM (control), TCM and GF-dep-TCM. TCM disrupted EC junctions while GF-dep-TCM did not because of the absence of hVEGF165. Scale bar, 50 μm. (h) Anti-ZO-1 (green) antibody and anti-phalloidin (red) staining. GF-dep-TCM-conditioned LEC-CM (GF-dep-TCM-LEC) promoted disruption of EC junction. This was blocked by anti-VEGF165antibody treatment. Scale bar, 50 μm. Data (a,d) are reported as mean±s.e.m. Figure 4: GF-dep-TCM promote LN angiogenesis and enhance lung vascular permeability. ( a ) In the proliferation assays, 2,000 HUVECs per well were plated in 96-well plates and allowed to adhere overnight. On the following day, the media were exchanged with LEC-CM (cond. media), EGM or SFM. Three days later, proliferating cells were quantified at 450 nm by using the WST-1 reagent (* P =0.039, n =6). In the migration assays, 180 μl of EGM-2 or SFM or MB231-LEC-CM were added to the bottom chambers (CIM-plates), HUVECs (45,000 cells per well) were added to the top chamber. The bottom and top chambers were combined, loaded in the RTCA system and the cell index was measured continuously at 20 h (* P =0.011, n =2). In adhesion assays, HUVECs (25,000 cells per well) in 100 μl of EGM-2 or SFM or MB231-LEC-CM were added in E-plates, after which the plate was loaded into the RTCA system. Cell indices at 3 h were analysed (* P =0.042 at 3 h, n =2). ( b ) HUVEC and LEC tube formation (at 20 h) was induced by MB231-LEC-CM in matrigel matrix. Scale bar, 200 μm. ( c ) Human growth factor (hVEGF 165 /hEGF)-depleted TCM (GF-dep-TCM) or SFM were subcutaneously administered daily for 10 days, the nude mice were killed and brachial LNs (Br-LNs) were excised and analysed with anti-mouse CD31 antibodies (green). Scale bar, 1 mm. ( d ) Quantification of c (* P =0.032, n =12). ( e ) Br-LNs from GF-dep-TCM-treated animals were probed with anti-mVEGF 164 (green); mLV (red). Scale bar, 500 μm. ( f ) GF-dep-TCM-treated animals were perfused with FITC-dextran (70 kDa) 1 h before termination. Collected lungs were stained with anti-mCD31 (red); dextran (green). Scale bar, 1,000 μm. ( g ) Anti-ZO-1 antibody staining (green) of HUVEC monolayers treated with SFM (control), TCM and GF-dep-TCM. TCM disrupted EC junctions while GF-dep-TCM did not because of the absence of hVEGF 165 . Scale bar, 50 μm. ( h ) Anti-ZO-1 (green) antibody and anti-phalloidin (red) staining. GF-dep-TCM-conditioned LEC-CM (GF-dep-TCM-LEC) promoted disruption of EC junction. This was blocked by anti-VEGF 165 antibody treatment. Scale bar, 50 μm. Data ( a , d ) are reported as mean±s.e.m. Full size image After treating animals with GF-dep-TCM or SFM, brachial LNs were probed with anti-mCD31 antibodies ( Fig. 4c ). LNs from GF-dep-TCM-treated mice showed enhanced angiogenesis ( Fig. 4d ). mVEGF 164 was detected around mLVs in the GF-dep-TCM-treated LNs ( Fig. 4e ), but not in SFM-treated LNs. mVEGF 164 was not found in the αSMA-positive area, but colocalized with mLVs ( Supplementary Fig. 14b ). To measure lung vascular permeability, FITC-dextran (70 kDa) was intravenously injected after tumour conditioning: extravasation of dextran into the lungs was facilitated by GF-dep-TCM treatment ( Fig. 4f ). In vitro , although TCM disrupted the integrity of EC junctions of a HUVEC monolayer compared with SFM-treated controls, GF-dep-TCM did not cause junction disruption ( Fig. 4g ), consistent with hVEGF 165 depletion above ( Supplementary Fig. 13a ). However, CM prepared from LECs treated with GF-dep-TCM (‘GF-dep-TCM-LECs’) caused EC junction disruption in vitro , and anti-hVEGF 165 treatment normalized it ( Fig. 4h ). We confirmed that the junction disruption was not caused by EC apoptosis using cleaved-caspase 3 antibodies ( Supplementary Fig. 13c ). Anti-mVEGF 164 treatment inhibits lung and LN metastasis Lungs from GF-dep-TCM- or SFM-treated animals were probed with anti-human VEGF165 and anti-mouse VEGF164 antibodies ( Supplementary Fig. 14c ). Anti-mouse VEGF164 antibodies have very limited cross-reactivity to human VEGF 165 (<0.04% according to R&D systems for the anti-VEGF 164 antibody AF-493-NA). hVEGF165 was not detected in either group, but mVEGF164 was detected around the mLVs in GF-dep-TCM-treated lungs, demonstrating that TCM lacking hVEGF 165 (white) influences the mLVs to express mVEGF164 (green; Supplementary Fig. 14c ). GF-dep-TCM-treated animals were systemically administered anti-mVEGF 164 or anti-hVEGF 165 antibodies (5 mg kg −1 , intraperitoneal (i.p. ), every 4 days) during the GF-dep-TCM induction phase. We discovered that anti-mVEGF164 treatment normalized vascular permeability in GF-dep-TCM-treated lungs, whereas anti-hVEGF 165 did not ( Fig. 5a ). 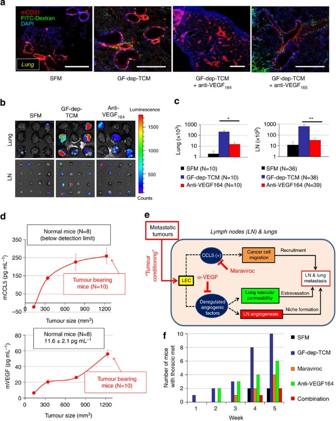Figure 5: Anti-mVEGF164and maraviroc treatment inhibits LN and lung metastasis. (a) Nude mice were treated with GF-dep-TCM or SFM for 2 weeks. In addition, anti-hVEGF165or and anti-mVEGF164antibodies (i.p. injection, 5 mg kg−1, at days 1, 5, 10, 14) were administered. FITC-dextran perfusion showed that lung vascular permeability was increased by GF-dep-TCM treatment. The increased permeability was normalized not by anti-hVEGF165but by anti-mVEGF164. Scale bar, 1,000 μm. (b) Based on the result ina, we administered anti-mVEGF164antibodies to inhibit GF-dep-TCM-induced metastasis. Nude mice were treated with SFM or GF-dep-TCM or GF-dep-TCM+Anti-mVEGF164antibodies for 2 weeks (i.p. injection, 5 mg kg−1, at days 1, 5, 10, 14). After 2 weeks, luc-MB231 tumour cells were orthotopically inoculated in the inguinal mammary fat pads. After 5 weeks of tumour inoculation, LNs and lungs were excised, incubated in D-luciferin solution and imaged under the IVIS imager. (c) Averaged photon flux in the lungs (n=10) and LNs (n=36–39) was quantified by using Living Image 3D Analysis (Xenogen; *P=0.033, **P=0.006). (d) Plasma concentration of mCCL5 and mVEGF in mice with and without MB231 tumours (n=8–10). Mouse plasma was obtained at 2, 3, 4 and 5 weeks after tumour inoculation. At week 5, when the tumour size was around 1,200 mm3, the plasma concentration of mCCL5 and mVEGF was ~260 and 56 pg ml−1, respectively (n=3). (e) Conceptual figure of tumour-conditioned LECs mediated LN and lung metastasis. Tumour-conditioned LECs express CCL5, which induces tumour cell recruitment, and VEGF, which promotes angiogenesis and tumour extravasation. Blocking each target inhibits LN and lung metastasis. (f) Dual inhibition of VEGF and the CCL5-CCR5 axis. There are five groups described: not conditioned (SFM treated), tumour conditioned (GF-dep-TCM), maraviroc treated, anti-mVEGF164treated and combination group. We treated with anti-mVEGF164antibodies (i.p. injection, 5 mg kg−1per 4 days) during GF-dep-TCM induction; maraviroc (8 mg kg−1per day, p.o.) after two weeks of GF-dep-TCM induction until the end of the experiment (n=10). Data (c,d) are reported as mean±s.e.m. Figure 5: Anti-mVEGF 164 and maraviroc treatment inhibits LN and lung metastasis. ( a ) Nude mice were treated with GF-dep-TCM or SFM for 2 weeks. In addition, anti-hVEGF 165 or and anti-mVEGF 164 antibodies (i.p. injection, 5 mg kg −1 , at days 1, 5, 10, 14) were administered. FITC-dextran perfusion showed that lung vascular permeability was increased by GF-dep-TCM treatment. The increased permeability was normalized not by anti-hVEGF 165 but by anti-mVEGF 164 . Scale bar, 1,000 μm. ( b ) Based on the result in a , we administered anti-mVEGF 164 antibodies to inhibit GF-dep-TCM-induced metastasis. Nude mice were treated with SFM or GF-dep-TCM or GF-dep-TCM+Anti-mVEGF 164 antibodies for 2 weeks (i.p. injection, 5 mg kg −1 , at days 1, 5, 10, 14). After 2 weeks, luc-MB231 tumour cells were orthotopically inoculated in the inguinal mammary fat pads. After 5 weeks of tumour inoculation, LNs and lungs were excised, incubated in D-luciferin solution and imaged under the IVIS imager. ( c ) Averaged photon flux in the lungs ( n =10) and LNs ( n =36–39) was quantified by using Living Image 3D Analysis (Xenogen; * P =0.033, ** P =0.006). ( d ) Plasma concentration of mCCL5 and mVEGF in mice with and without MB231 tumours ( n =8–10). Mouse plasma was obtained at 2, 3, 4 and 5 weeks after tumour inoculation. At week 5, when the tumour size was around 1,200 mm 3 , the plasma concentration of mCCL5 and mVEGF was ~260 and 56 pg ml −1 , respectively ( n =3). ( e ) Conceptual figure of tumour-conditioned LECs mediated LN and lung metastasis. Tumour-conditioned LECs express CCL5, which induces tumour cell recruitment, and VEGF, which promotes angiogenesis and tumour extravasation. Blocking each target inhibits LN and lung metastasis. ( f ) Dual inhibition of VEGF and the CCL5-CCR5 axis. There are five groups described: not conditioned (SFM treated), tumour conditioned (GF-dep-TCM), maraviroc treated, anti-mVEGF 164 treated and combination group. We treated with anti-mVEGF 164 antibodies (i.p. injection, 5 mg kg −1 per 4 days) during GF-dep-TCM induction; maraviroc (8 mg kg −1 per day, p.o.) after two weeks of GF-dep-TCM induction until the end of the experiment ( n =10). Data ( c , d ) are reported as mean±s.e.m. Full size image Next, the anti-mVEGF 164 antibody was tested in GF-dep-TCM-induced metastasis models like the one discussed above induced by complete TCM ( Fig. 2 ). Five weeks after tumour inoculation in the induced mice, lungs and LNs were collected to assess metastases ex vivo ( Fig. 5b ). Anti-VEGF 164 antibody inhibited metastasis in the LNs and lungs ( Fig. 5b,c ), demonstrating that lung vascular remodelling and LN angiogenesis are initiated by GF-dep-TCM-induced VEGF, and the blockade of the VEGF function prevents metastatic extravasation and colonization. Dual inhibition of CCR5/VEGF strongly blocks metastasis We established MB231 tumour xenografts ( n =10) without TCM pretreatment, and collected plasma at 2, 3, 4 and 5 weeks to estimate human tumour xenograft-induced mouse VEGF and mCCL5 expression ( Fig. 5d ). Plasma samples from normal mice without tumours ( n =8) were used as controls. Plasma concentration of mCCL5 and mVEGF was increased as tumours grew, compared with normal mice: mCCL5 plasma concentration was 259.2±43.6 pg ml −1 , and mVEGF was 56.1±4.9 pg ml −1 when the mean tumour volume was 1,232±223 mm 3 (week 5). We hypothesized that dual inhibition of CCR5 and VEGF signalling would inhibit metastasis more effectively than single inhibition of each target, as the mCCL5 and mVEGF function as tumour recruitment factor and colonization factor, respectively ( Fig. 5e ). We carried out dual inhibition of CCR5 and VEGF as described in Supplementary Fig. 15 . We observed that 60% of the mice had metastases in the anti-mVEGF 164 group, 40% had metastases in the maraviroc group and only 20% had metastases in the combination group. All the mice (100%) had thoracic metastasis in the no-treatment group ( Fig. 5f ). The IL6-Stat3 axis induces CCL5 expression in LECs We next identified key targets in tumour-conditioned LECs, which are specifically phosphorylated by TCM treatment. Among 46 kinase phosphorylation sites screened, both S727 and Y705 of Stat3 were exclusively phosphorylated in LECs by TCM treatment ( Fig. 6a ). The presence of phospho-Stat3 (pStat3: Y705) in TCM-treated LECs was confirmed in separate western blots ( Fig. 6b ). Importantly, the essential role of pStat3 in CCL5 expression in LECs was confirmed by using a small molecule, Stattic, an inhibitor of phosphorylation and dimerization of Stat3 (ref. 13 ) ( Fig. 6c,d ). We next showed that IL6 and granulocyte–macrophage colony-stimulating factor (GM-CSF) are exclusively expressed in TNBC cell lines (MB231 and SUM149), but not in MCF7 or LECs ( Fig. 6e,f ). GM-CSF was not considered as a key cytokine in the metastatic process because GM-CSF is known to phosphorylate Stat5 [14] and we saw no pStat5 in TCM-treated LECs ( Fig. 6a ). Human IL6 in MB231/SUM149/MCF7-TCM and LEC-CM was measured by ELISAs. High levels of IL6 were only seen in the TNBC cell lines ( Fig. 6g ). Only TCM containing IL6-induced pStat3 in LECs and IL6-dep-TCM (TCM immunodepleted of IL6) failed to induce phosphorylation of Stat3 in LECs ( Fig. 6h ; Supplementary Fig. 16a,b,d ). These data demonstrate that TNBC cell-secreted IL6 is the crucial factor for induction of Stat3 phosphorylation in LECs. We also showed that the IL6-gp130-Jak2-Stat3 axis is critical for IL6 signal transduction ( Supplementary Fig. 17 ). In functional assays, IL6-dep-TCM did not induce CCL5 expression in LECs compared with intact TCM, but still induced some VEGF expression ( Fig. 6i ). These results show that CCL5 expression in MB231-LECs is totally IL6 driven, but VEGF expression can be induced by IL6 and other unknown factors in the TCM. 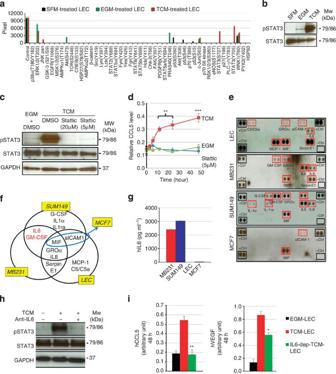Figure 6: Tumour cell-secreted IL6 phosphorylates Stat3, which induces CCL5 and VEGF expression in LECs. (a) Reverse western assays with the human phospho-kinase antibody arrays (R&D systems) simultaneously detected the relative amounts of 46 phosphorylation sites in LECs. We compared the effects of SFM, EGM and TCM treatment in LECs (overnight incubation). (b) Phosphorylation of Stat3 in TCM-treated LECs was assessed in a separate western blot. (c) Phosphorylation of Stat3 was completely blocked by Stattic (5, 20 μM) in LECs. GAPDH was used as a loading control. (d) CCL5 levels were assessed by ELISA following 5 μM Stattic treatment (**P<0.01, ***P=0.0008,n=4). (e) Reverse western assays with the human cytokine antibody arrays (R&D systems) detected the relative amounts of 36 cytokines in MB231, SUM149, MCF7 and LEC-CM. Representative images of the cytokine array membranes. (f) Summary of the cytokine array results ine. IL6 and GM-CSF were expressed only in TNBC cell lines (MB231 and SUM149). (g) ELISA was used to determine levels of IL6 in MB231 and SUM149 cells (n=3). (h) Stat3 phosphorylation was assessed in the presence or absence of anti-IL6 in LECs. GAPDH was used as a loading control. (i) CCL5 and VEGF expression was measured by ELISA in the presence or absence of anti-IL6 in LECs. VEGF expression was significantly reduced by IL6 depletion, but not completely (**P=0.0075, *P=0.032,n=3). Data (a,d,g,i) are reported as mean±s.e.m. Original gel images of data (b,c,h) are presented inSupplementary Fig. 25. Figure 6: Tumour cell-secreted IL6 phosphorylates Stat3, which induces CCL5 and VEGF expression in LECs. ( a ) Reverse western assays with the human phospho-kinase antibody arrays (R&D systems) simultaneously detected the relative amounts of 46 phosphorylation sites in LECs. We compared the effects of SFM, EGM and TCM treatment in LECs (overnight incubation). ( b ) Phosphorylation of Stat3 in TCM-treated LECs was assessed in a separate western blot. ( c ) Phosphorylation of Stat3 was completely blocked by Stattic (5, 20 μM) in LECs. GAPDH was used as a loading control. ( d ) CCL5 levels were assessed by ELISA following 5 μM Stattic treatment (** P <0.01, *** P =0.0008, n =4). ( e ) Reverse western assays with the human cytokine antibody arrays (R&D systems) detected the relative amounts of 36 cytokines in MB231, SUM149, MCF7 and LEC-CM. Representative images of the cytokine array membranes. ( f ) Summary of the cytokine array results in e . IL6 and GM-CSF were expressed only in TNBC cell lines (MB231 and SUM149). ( g ) ELISA was used to determine levels of IL6 in MB231 and SUM149 cells ( n =3). ( h ) Stat3 phosphorylation was assessed in the presence or absence of anti-IL6 in LECs. GAPDH was used as a loading control. ( i ) CCL5 and VEGF expression was measured by ELISA in the presence or absence of anti-IL6 in LECs. VEGF expression was significantly reduced by IL6 depletion, but not completely (** P =0.0075, * P =0.032, n =3). Data ( a , d , g , i ) are reported as mean±s.e.m. Original gel images of data ( b , c , h ) are presented in Supplementary Fig. 25 . Full size image To establish the relevance of these results to human disease, we analysed The Cancer Genome Atlas (TCGA) mRNA-sequencing data from TNBC and estrogen receptor+/progesterone receptor+/human epidermal growth factor receptor 2− (ER+/PR+/HER2−) tumours and discovered higher levels of expression of IL6 and CCL5 in TNBC ( Supplementary Fig. 18a,b ). Moreover, IL6 and CCL5 are significantly associated with LN-positive breast cancer in TNBC ( Supplementary Fig. 18c,d ), suggesting that the IL6-CCL5 axis that we discovered has clinical relevance for metastatic breast cancer patients. pStat3-pc-Jun-pATF-2 complex and HIF1α express CCL5/VEGF We observed that Stattic inhibited IL6-induced CCL5 and VEGF expression in LECs; SP600125, a c-Jun N-terminal kinase inhibitor, blocked IL6-induced expression of CCL5 but not of VEGF in LECs ( Fig. 7a ). Western blots showed that c-Jun and ATF-2 were constitutively phosphorylated in LECs, while Stat3 phosphorylation required IL6 ( Fig. 7b ). SP600125 reduced the amount of pc-Jun and pATF-2 but pStat3 was not affected. With Stattic, pStat3 disappeared but pc-Jun and pATF-2 were maintained ( Fig. 7b ). We next performed co-immunoprecipitation with LEC nuclear extracts. Strikingly, pStat3, pc-Jun and pATF-2 form a ternary complex in response to IL6 treatment ( Fig. 7c ). After treating with SP600125 or Stattic, the complexes disappeared ( Fig. 7c ). 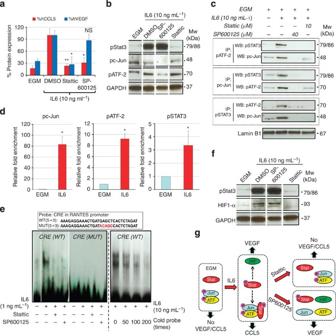Figure 7: The pStat3-pc-Jun-pATF-2 ternary complex is central for CCL5 expression and pStat3-dependent HIF-1α induces VEGF expression. (a) CCL5/VEGF expression in IL6-treated LEC. LEC were treated with EGM, IL6 only or IL6 with inhibitors (Stattic, stat3 inhibitor; SP600125, JNK inhibitor). IL6-dependent CCL5/VEGF expression was assessed using ELISAs. CCL5 with Stattic (**P=0.009,n=3); CCL5 with SP600125 (*P=0.028,n=3), VEGF with Stattic (*P=0.041,n=3). (b) Western blot assays with LEC, EGM activated pc-Jun and pATF-2 but not pStat3; only IL6 treatment induced pStat3. SP600125 blocked pc-Jun and pATF-2 while Stattic selectively blocked pStat3. (c) Co-immunoprecipitation assays with nuclear extracts. Lamin B1 was used as a nuclear extract loading control. (d) ChIP assays, real-time PCR analysis of recruitment of pATF-2, pc-Jun and pStat3 to the CRE region (site 2) of CCL5 promoter with IL6 (10 ng ml−1) treatment (*P<0.05,n=3). (e) The two strands of the wild-type CRE oligonucleotide and of mutated CRE conjugated with biotin were synthesized (Invitrogen). For the binding reaction, 3mg nuclear extract and 0.5mg poly(dI-dC) with or without excess unlabelled CRE oligonucleotide were incubated in binding buffer for 10min at RT, after which oligonucleotide-biotin was added and incubated for 30 min at RT. Ten microlitres of binding sample was mixed with TBE sample buffer (Invitrogen), loaded on the gel and run for 1h at 120V in 0.5 TBE running buffer. The gel was transferred to a DNA transfer stack (Invitrogen). The nylon membrane was dried and cross-linked under a UV source (305nm) for 15min, then probed by the Chemiluminescent Nucleic Acid Detection Module (Pierce). (f) HIF-1α and pStat3 levels were assessed by western blot in the presence of IL6 treatment. (g) Graphical summary. pc-Jun-pATF-2 binary complexes and unphosphorylated Stat3 are present in n-LECs but there is no CCL5/VEGF expression. IL6 induces Stat3 phosphorylation and activates formation of the pStat3-pc-Jun-pATF-2 ternary complex, which is essential for CCL5 expression. pStat3 promotes HIF-1α expression and separately induces VEGF expression. On Stattic treatment, pStat3 and the ternary complex disappear, resulting in no expression of CCL5 and VEGF; the pc-Jun-pATF-2 binary complex that remains on Stattic treatment does not induce either CCL5 or VEGF expression. SP600125 dissociates both ternary and binary complexes, but pStat3 separately induces HIF-1α and VEGF expression. Data (a,d) are reported as mean±s.e.m. Original gel images of data (b,c,f) are presented inSupplementary Fig. 25. NS, nonsignificant. Figure 7: The pStat3-pc-Jun-pATF-2 ternary complex is central for CCL5 expression and pStat3-dependent HIF-1α induces VEGF expression. ( a ) CCL5/VEGF expression in IL6-treated LEC. LEC were treated with EGM, IL6 only or IL6 with inhibitors (Stattic, stat3 inhibitor; SP600125, JNK inhibitor). IL6-dependent CCL5/VEGF expression was assessed using ELISAs. CCL5 with Stattic (** P =0.009, n =3); CCL5 with SP600125 (* P =0.028, n =3), VEGF with Stattic (* P =0.041, n =3). ( b ) Western blot assays with LEC, EGM activated pc-Jun and pATF-2 but not pStat3; only IL6 treatment induced pStat3. SP600125 blocked pc-Jun and pATF-2 while Stattic selectively blocked pStat3. ( c ) Co-immunoprecipitation assays with nuclear extracts. Lamin B1 was used as a nuclear extract loading control. ( d ) ChIP assays, real-time PCR analysis of recruitment of pATF-2, pc-Jun and pStat3 to the CRE region (site 2) of CCL5 promoter with IL6 (10 ng ml −1 ) treatment (* P <0.05, n =3). ( e ) The two strands of the wild-type CRE oligonucleotide and of mutated CRE conjugated with biotin were synthesized (Invitrogen). For the binding reaction, 3mg nuclear extract and 0.5mg poly(dI-dC) with or without excess unlabelled CRE oligonucleotide were incubated in binding buffer for 10min at RT, after which oligonucleotide-biotin was added and incubated for 30 min at RT. Ten microlitres of binding sample was mixed with TBE sample buffer (Invitrogen), loaded on the gel and run for 1h at 120V in 0.5 TBE running buffer. The gel was transferred to a DNA transfer stack (Invitrogen). The nylon membrane was dried and cross-linked under a UV source (305nm) for 15min, then probed by the Chemiluminescent Nucleic Acid Detection Module (Pierce). ( f ) HIF-1α and pStat3 levels were assessed by western blot in the presence of IL6 treatment. ( g ) Graphical summary. pc-Jun-pATF-2 binary complexes and unphosphorylated Stat3 are present in n-LECs but there is no CCL5/VEGF expression. IL6 induces Stat3 phosphorylation and activates formation of the pStat3-pc-Jun-pATF-2 ternary complex, which is essential for CCL5 expression. pStat3 promotes HIF-1α expression and separately induces VEGF expression. On Stattic treatment, pStat3 and the ternary complex disappear, resulting in no expression of CCL5 and VEGF; the pc-Jun-pATF-2 binary complex that remains on Stattic treatment does not induce either CCL5 or VEGF expression. SP600125 dissociates both ternary and binary complexes, but pStat3 separately induces HIF-1α and VEGF expression. Data ( a , d ) are reported as mean±s.e.m. Original gel images of data ( b , c , f ) are presented in Supplementary Fig. 25 . NS, nonsignificant. Full size image The cAMP-responsive element (CRE) in the promoter of the CCL5 gene is known to regulate its expression in alveolar epithelial cells [15] . ATF-2 binds to the CRE [16] . Moreover, c-Jun and ATF-2 have been observed in a binary complex [17] . Importantly, Stat3 can interact with c-Jun and participate in cooperative transcriptional activation [18] . We hypothesized that the pStat3-pc-Jun-pATF-2 ternary complex would bind to the CRE site in CCL5 promoter. To test this hypothesis, we performed chromatin immunoprecipitation (ChIP) assay with ~200-base pair chromatin fragments by sonication of LECs treated with IL6 (10 ng ml −1 ; Fig. 7d ; Supplementary Fig. 19 ). Three regions of the CCL5 promoter with the CRE site (−316 to −69 bp) and two distal sites (−1,064 to −815 and −474 to −711 bp) were tested ( Supplementary Fig. 19a ). We found that pStat3-pc-Jun-pATF−2 ternary complex specifically bound to only the CRE site (site 2) by real-time quantitative PCR. In contrast, the distal sites (sites 1 and 3) do not show significant complex-binding capabilities ( Supplementary Fig. 19b,c ). Compared with vehicle treatment, ChIPs on LECs with IL6 treatment showed specific pStat3-pc-Jun-pATF-2 ternary complex enrichment for binding to this region ( Fig. 7d ). In addition, electrophoretic mobility shift assays (EMSAs) were performed to show binding between the ternary complex and the CRE oligonucleotide ( Fig. 7e ). When LECs were treated with IL6, nuclear proteins bound to the CRE oligonucleotide; however, Stattic or SP600125 treatment inhibited the binding. No binding was observed on the mutated CRE, and excess unlabelled CRE oligonucleotide competitively inhibited the binding ( Fig. 7e ). VEGF expression in TCM-treated LECs can be triggered by multiple signalling pathways, since IL6 depletion did not completely inhibit VEGF expression ( Fig. 6i ). However, we observed that IL6 promoted the expression of HIF-1α in LECs ( Fig. 7f ), and this expression was blocked by Stattic but not by SP600125, demonstrating that HIF-1α expression is pStat3 dependent, but not associated with pc-Jun or pATF-2. Summarizing these immunoblot results ( Fig. 7b–f ) and VEGF/CCL5 expression data ( Fig. 7a ), we can conclude that the IL6-induced pStat3-pc-Jun-pATF-2 ternary complex is essential for CCL5 expression; VEGF expression is pStat3 induced and possibly HIF-1α associated and does not require pc-Jun or pATF-2 ( Fig. 7g ). Targeting of IL6 and pStat3 blocks LN and lung metastasis The mechanistic results above indicate that the IL6-Stat3 axis is a key inducer of CCL5 and VEGF expression in LECs. Thus, we tried to inhibit GF-dep-TCM-induced metastasis by targeting IL6 and pStat3 as described in Supplementary Fig. 20b . We generated GF/IL6-dep-TCM by immunodepleting IL6 from GF-dep-TCM. Separately, we chose S3I-201, another pStat3 inhibitor with the same mechanism of action as Stattic; S3I-201 has been tested in vivo [19] . We showed that S3I-201 inhibited pStat3 levels in IL6-treated LECs ( Supplementary Fig. 20a ). All mice pretreated with GF-dep-TCM for 2 weeks before tumour inoculation developed metastases at 5 weeks; 44% of the mice (4/9) treated with S3I-201 during the pretreatment phase developed metastases, only 22% (2/9) of the mice pretreated with GF/IL6-dep-TCM had metastases that was less than the 33% (3/9) of mice with metastases in the SFM-treated group ( Fig. 8a ). We observed significant reductions in lung and LN metastases by IVIS imaging, macroscopic morphology and anti-cytokeratin immunostaining ( Fig. 8b,c ; Supplementary Fig. 20c ). Tumour size was not influenced by these treatments ( Supplementary Fig. 20d ). The mechanisms presented in this study are summarized in the schematic ( Fig. 8d ). 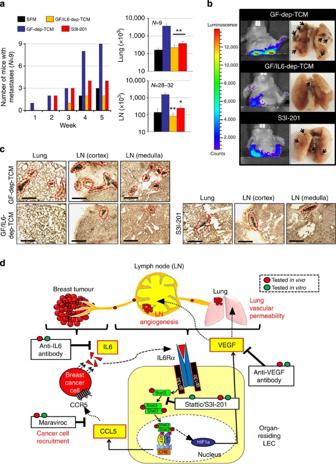Figure 8: Inhibition of IL6 and pStat3 blocks GF-dep-TCM-induced LN and lung metastasis. (a) There are four groups described: SFM treated, tumour conditioned (GF-dep-TCM), tumour conditioned without IL6 and pStat3 inhibited (by using a pStat3 inhibitor, ‘S3I-201’). After 2 weeks of these treatments, inguinal primary tumour was established, and thoracic metastasis was monitored for 5 weeks (as described inSupplementary Fig. 20b). The number of mice in each group with thoracic metastasis is shown. Lung metastasis was blocked by both IL6 depletion and S3I–201 treatment (n=9, **P<0.01). LN metastasis was blocked by IL6 depletion and by S3I–201 treatment (n=28–32, *P=0.027, **P=0.0007). (b) Representative images of live animals in the IVIS imager, and images of collected lungs. Black arrows represent tumour nodules. (c) Immunohistochemistry with anti-cytokeratin antibodies on the lungs and LNs (cortex and medulla). Metastatic colonies are delineated with red-dotted curves. Scale bar, 500 μm. (d) Graphical summary of the whole study. Breast cancer cells secrete IL6 that interacts with IL6 receptor on LECs within the lungs and LNs. Activated IL6 receptors transduce the signals through gp130, phosphorylating lymphatic Stat3. pStat3 translocates into the nucleus to form the pStat3-pc-Jun-pATF-2 ternary complex, which is essential for CCL5 expression by targeting the CRE region in its promoter. pStat3 also induces HIF-1α to ultimately express VEGF in LECs. LEC-secreted CCL5 recruits CCR5-positive breast cancer cells into the lymphatic system. The secreted VEGF enhances lung vascular permeability and induces LN angiogenesis to promote metastatic extravasation and colonization. The four possible targets in the overall mechanism were blocked as follows: by anti-IL6 antibody (to target IL6), by maraviroc (to interrupt the CCL5-CCR5 axis), by anti-VEGF antibody (to block LN angiogenesis and lung vascular leakiness) and by Stattic/S3I-201 (to inhibit pStat3). Treatments are marked with red and green circles, which represent ‘testedin vivo’ and ‘testedin vitro’ respectively. Figure 8: Inhibition of IL6 and pStat3 blocks GF-dep-TCM-induced LN and lung metastasis. ( a ) There are four groups described: SFM treated, tumour conditioned (GF-dep-TCM), tumour conditioned without IL6 and pStat3 inhibited (by using a pStat3 inhibitor, ‘S3I-201’). After 2 weeks of these treatments, inguinal primary tumour was established, and thoracic metastasis was monitored for 5 weeks (as described in Supplementary Fig. 20b ). The number of mice in each group with thoracic metastasis is shown. Lung metastasis was blocked by both IL6 depletion and S3I–201 treatment ( n =9, ** P <0.01). LN metastasis was blocked by IL6 depletion and by S3I–201 treatment ( n =28–32, * P =0.027, ** P =0.0007). ( b ) Representative images of live animals in the IVIS imager, and images of collected lungs. Black arrows represent tumour nodules. ( c ) Immunohistochemistry with anti-cytokeratin antibodies on the lungs and LNs (cortex and medulla). Metastatic colonies are delineated with red-dotted curves. Scale bar, 500 μm. ( d ) Graphical summary of the whole study. Breast cancer cells secrete IL6 that interacts with IL6 receptor on LECs within the lungs and LNs. Activated IL6 receptors transduce the signals through gp130, phosphorylating lymphatic Stat3. pStat3 translocates into the nucleus to form the pStat3-pc-Jun-pATF-2 ternary complex, which is essential for CCL5 expression by targeting the CRE region in its promoter. pStat3 also induces HIF-1α to ultimately express VEGF in LECs. LEC-secreted CCL5 recruits CCR5-positive breast cancer cells into the lymphatic system. The secreted VEGF enhances lung vascular permeability and induces LN angiogenesis to promote metastatic extravasation and colonization. The four possible targets in the overall mechanism were blocked as follows: by anti-IL6 antibody (to target IL6), by maraviroc (to interrupt the CCL5-CCR5 axis), by anti-VEGF antibody (to block LN angiogenesis and lung vascular leakiness) and by Stattic/S3I-201 (to inhibit pStat3). Treatments are marked with red and green circles, which represent ‘tested in vivo ’ and ‘tested in vitro ’ respectively. Full size image According to the ‘seed and soil hypothesis’, metastatic cancer cells function as ‘seeds’ and a particular organ microenvironment serves as the ‘soil’ [20] . It is difficult for cancer cells (‘seeds’) to survive outside their site of origin, thus they have to find a suitable location (‘soil’) where they can settle and grow. They also manipulate the microenvironment to optimize these pre-metastatic locations [21] . In this study, we show for the first time that tumour cell-secreted IL6 conditions LECs in the pre-metastatic organs to prime them and promotes breast cancer metastasis. Paracrine signals regulated by the IL6-Stat3 axis and operating between cancer cells and LECs play a crucial role in the induction of CCL5 and VEGF expression in LECs within pre-metastatic organs facilitating tumour cell recruitment, extravasation and colonization ( Fig. 8d ). IL6 is an inflammatory cytokine that leads to activation of the Jak family and glycoprotein 130 (gp130) to phosphorylate Stat3 on interaction with the IL6 receptors [22] . In our experiment using LECs, we showed that gp130, Jak2 and Stat3 were phosphorylated by TCM containing IL6 ( Supplementary Fig. 17 ). Stat3 is a transcription factor that contributes to the expression of diverse cytokines, chemokines and growth factors [23] , [24] . Thus, the IL6-Stat3 axis has been explored in cancer [25] , [26] , [27] . The IL6-Stat3 axis promotes tumorigenesis [28] , [29] , [30] , [31] , causes chemoresistance [32] , [33] , [34] , [35] , [36] and contributes to epithelial–mesenchymal transition [37] , [38] , [39] . IL6-Stat3 feed-forward loops amplify pro-tumorigenic and pro-metastatic signals in cancer cells [40] , [41] . However, the role and importance of the IL6-Stat3 axis in LECs has not been studied before. We document that LECs can be actively involved in breast tumour metastasis as one of the orchestrators of metastasis via the IL6-Stat3 axis. We show that TCM containing IL6 induces lymphatic expression of CCL5 in the pre-metastatic organs, forming chemotactic gradients to recruit CCR5-positive cancer cells into the organs ( Figs 1 and 2 ). We measured the concentration of mCCL5 in the plasma of mice treated with TCM over a 2-week period ( Supplementary Fig. 3 ). mCCL5 increased with time of TCM treatment, and the increasing trend was sustained for an additional week after stopping the TCM treatment (maximum level=450 pg ml −1 ). Compared with the level of mCCL5 (250 pg ml −1 ) in normal tumour xenograft models without TCM treatment ( Fig. 5d ), TCM pretreatment can create a dramatic CCL5 gradient in the system to facilitate tumour dissemination. TCM-induced metastasis was blocked by maraviroc, a CCR5 inhibitor ( Fig. 2 ). We also evaluated the therapeutic effects of maraviroc in spontaneous metastasis models without TCM ( Supplementary Fig. 9 ). Maraviroc treatment inhibited tumour metastasis, suggesting that the CCL5-CCR5 axis is also central in general and spontaneous metastasis models. The CCL5-CCR5 axis needs to be further investigated in murine tumour models as well, since our nude mouse models may have limitations with the absence of T lymphocytes that could be one of the mediators of metastasis. To establish the clinical relevance of our findings, we evaluated the IL6-CCL5 axis by analysing TCGA mRNA-sequencing data sets ( Supplementary Fig. 18 ). Both IL6 and CCL5 were significantly overexpressed in TNBC tumours over ER+/PR+/HER2− tumours ( Supplementary Fig. 18a,b ). This finding is consistent with our results that only TNBC cell lines (MB231 and SUM149) express IL6 and induce CCL5 expression in LECs and that the MCF7 cell line does not ( Figs 1d and 6g ). In addition, the expression of IL6 and CCL5 mRNAs was significantly correlated in LN-positive TNBC samples over LN-negative samples, suggesting that the IL6 and CCL5 can serve as therapeutic and prognostic markers in TNBC metastasis ( Supplementary Fig. 18c ). The axis needs to be further studied in other subtypes of breast cancer and other cancers to expand the application. To expand on the discovery that organ-residing LECs promote metastasis via CCL5 expression ( Figs 1 and 2 ), we examined whether LECs exist in the primary tumours, as well to orchestrate metastasis by actually connecting the primary tumours and distant organs. LECs were detected in the MB231 tumours; moreover, LECs within the tumour expressed CCL5 ( Supplementary Fig. 21 ). This suggests that LECs can form a CCL5 gradient even in tumour stroma, which can trigger initial recruitment of cancer cells into the lymphatic system via intratumoural and peritumoural LVs. The presence of LECs in the tumour is due to tumour lymphangiogenesis, driven by tumour cell-secreted lymphangiogenic factors such as VEGF-C/D [42] , [43] . To expand on the classical understanding of tumour lymphangiogenesis, we add a new concept that LECs within tumours and distal organs can create chemotactic gradients to facilitate lymphogenous metastasis via the CCL5-CCR5 axis. We investigated mechanisms of CCL5 upregulation in LECs by TCM. In previous studies of CCL5 regulation, tumour-necrosis factor-α, not IL6/gp130, induced CCL5 expression in vascular smooth muscle cells [44] in an NFkB-dependent manner; NFkB-dependent CCL5 expression has also been studied in other types of cells [44] , [45] , [46] . In this study, however, we found that IL6-induced CCL5 is not colocalized with αSMA-positive cells ( Supplementary Fig. 2b ) and is not associated with an NFkB-Stat3 complex ( Supplementary Fig. 16c,d ). Instead, pStat3 forms a ternary complex consisting of pStat3, pc-Jun and pATF-2 in response to IL6, which regulates CCL5 expression in the lymphatic system; this mechanism has not been previously discovered. ChIP and EMSA experiments showed the binding of the ternary complex to the CRE site of the CCL5 promoter ( Fig. 7d,e ; Supplementary Fig. 19 ). We additionally tested the effect of EGF on CCL5 expression in LECs, as MB231-LECs express EGF ( Fig. 3g ) and EGF-derived Src pathways may contribute to activation of Stat3 pathways [29] . EGF treatment phosphorylated c-Jun and ATF-2, but not Stat3 in LECs, and did not induce CCL5 expression ( Supplementary Fig. 22 ). Interestingly, unlike LECs, HUVECs could not be conditioned by TCM ( Fig. 3g ; Supplementary Fig. 23 ). It has been reported that LECs express 3–4 times more gp130, compared with BEC [47] . Gp130 is a co-receptor of IL6 receptor and plays a role as an IL6 signal transducer [48] . We showed that the gp130-Jak2 axis is a pivotal bridge for IL6-pStat3 signalling transduction in LECs ( Supplementary Fig. 17 ), and consistently observed less gp130 as well as less pStat3 in BEC and no TCM effect ( Supplementary Fig. 23 ). Other molecular details of IL6-dependent induction of CCL5 remain to be elucidated. We showed that tumour-conditioned LECs also promote angiogenesis ( Figs 3 and 4 ), which has not been reported before. While physiological LECs maintain angiogenic homeostasis, the TCM-treated LEC secretome is abnormal and highly angiogenic. Breast cancer involves metastasis to the LNs, thus the LNs need to serve as metastatic niches [49] , [50] . One way tumours prime the LNs is by enhancing LN angiogenesis ensuring sufficient oxygen and nutrients around metastatic tumours [11] , [51] , [52] . We showed that LECs in the LNs are conditioned by TCM and induce LN angiogenesis ( Fig. 4c–e ). We observed that VEGF expression in TCM-induced LECs is partially IL6 driven ( Fig. 6i ). While IL6-depleted TCM did not induce any CCL5 in LECs, around 65% of total VEGF induced by TCM treatment was still expressed in LECs even in the absence of IL6. This demonstrates that molecules other than IL6 in the TCM, which we have not identified by our analysis, are also involved in metastasis by inducing angiogenesis; this needs to be further studied. We additionally studied recruitment of CD45-positive leukocytes and F4/80- or Iba1-positive macrophages to the lungs and LNs of TCM-treated animals ( Supplementary Figs 4 and 5 ). Importantly, these cells were not colocalized with TCM-induced mCCL5, suggesting that the infiltration of the macrophages or leukocytes is not triggered by mCCL5, and these cells do not express mCCL5 ( Supplementary Fig. 6 ). The recruitment of these leukocytes to the metastatic sites in TCM-treated animals could be caused by other unknown factors. We further hypothesized that macrophages can contribute to angiogenesis in the pre-metastatic organs, as macrophages are derived from monocytes that are differentiated from myeloid progenitor cells. Myeloid cells are one type of bone marrow-derived cells that are known to promote angiogenesis in the tumour microenvironment [53] . We investigated CD33-positive myeloid cells and assessed mVEGF 164 expression in the myeloid cells and LECs to dissect the relative angiogenic potentials of these cells. We found that both myeloid cells and LECs contribute to angiogenesis by expressing mVEGF 164 ( Supplementary Fig. 24 ). However, the myeloid cells were also not associated with CCL5 ( Supplementary Fig. 24 ). Thus, LECs play a key role in tumour cell recruitment through the CCL5-CCR5 axis and the pro-angiogenic phenotypes in the niches can be achieved by LECs and other cells like myeloid cells. On the basis of these findings, we tested several inhibitors in our metastasis models. We observed that anti-VEGF therapy prevented metastasis, and very surprisingly, the anti-VEGF treatment showed synergy with maraviroc treatment ( Fig. 5f ). This result suggests that current anti-angiogenic therapies can be combined with the Food and Drug Administration-approved anti-retroviral drug, maraviroc, which is orally available and safe for long-term use, giving rise to the possibilities for therapeutic intervention for metastatic breast cancer. We also targeted IL6 and pStat3 by using anti-IL6 antibodies and S3I-201, a pStat3 inhibitor. Both IL6 depletion and S3I-201 treatment inhibited LN and lung metastasis ( Fig. 8 ). This suggests that current anti-IL6 receptor therapy for rheumatoid arthritis (for example, tocilizumab) may improve metastatic breast cancer outcomes. Collectively, this study proposes a complex molecular crosstalk between TNBC cells and LECs in distal organs leading to enhanced metastasis and identifies the key players, IL6-Stat3, CCL5-CCR5 and VEGF ( Fig. 8d ), which can be targeted in a singular or combinatorial manner using repurposed drugs. Thus, this study has significant translational relevance. Cell culture HUVECs and LECs were purchased from Lonza, and grown in EGM-2 and EGM-2MV, respectively. MDA-MB-231, SUM149 and MCF7 breast cancer cells were gifts from Dr Zaver Bhujwalla (JHMI, Radiology and Oncology). MDA-MB-231-luc-D3H2LN was purchased from Caliper. MDA-MB-231, MDA-MB-231-luc-D3H2LN and MCF7 cells were propagated in RPMI-1640 medium supplemented with 10% fetal bovine serum (FBS) and 1% penicillin/streptomycin (Sigma). SUM149 cells were cultured in F-12 media supplemented with 5% FBS, 1 ng ml −1 hydrocortisone, 5 μg ml −1 insulin (Sigma) and 0.1 mM HEPES (Gibco). Conditioned media When MDA-MB-231, MCF7 and SUM149 cells reached confluence in T175 tissue culture flasks, the normal growth media were replaced with 8 ml SFM. After 24 h incubation, the supernatant was centrifuged and filtered through 0.2 μm syringe filters (Corning). The resulting TCM were stored in aliquots at −80 °C. When LECs/HUVECs reached 30–40% confluence in T75 tissue culture flasks, EGM were replaced with 30% TCM (TCM:EGM=3:7) to allow the TCM to condition the LECs/HUVECs. LECs/HUVECs were allowed to grow in the media for 3–4 days, then the media were replaced with 3 ml SFM with 2% FBS (not supplemented with bullet kit). After 48 h, the supernatant was centrifuged and filtered. The resulting tumour-conditioned LEC/HUVEC-CM (MB231-LECs or MB231-HUVECs) were stored in aliquots at −80 °C to avoid multiple freeze–thaws. Platypus cell migration assays Cancer cell migration was assessed by using the Oris cell migration kit (Platypus) [7] . MDA-MB-231 cells were pre-labelled with Cell Tracker Green (Invitrogen) according to the manufacturer’s protocol. Labelled cancer cells (50,000) in complete media (RPMI-1640) were added to each well of a 96-well plate containing stoppers to prevent the cells from settling in the centre region of the wells. Cells were allowed to adhere for 4 h, after which the stoppers were carefully removed. MB231-LEC-CM with or without inhibitors was added, and the cells that migrated to the centre of the well were quantified by measuring the fluorescence at 485/530 nm on a Victor V plate reader (Perkin Elmer). The migrated cells were visualized by imaging on the Eclipse T-100 fluorescence microscope (Nikon). Twenty micromoles of BX513 (Tocris), maraviroc (R&D Systems), SB328437 (Tocris) or anti-CCR7 antibodies (R&D systems, 30 μg ml −1 ) was used as inhibitor. ACEA cell migration/adhesion assays HUVEC migration was assessed using Cell Invasion/Migration plate (CIM-plates) (Roche) and the real-time cell analyzer (RTCA) system (ACEA Bioscience); adhesion was assessed using E-plate (Roche) in the RTCA system [54] . Briefly, the membrane of the top chamber of a CIM-plate was coated with fibronectin by adding 40 μl of 20 μg ml −1 fibronectin dissolved in phosphate-buffered saline (PBS) and incubating at 37 °C for 30 min. One hundred and eighty microlitres of EGM-2 (complete media for HUVECs) or EBM (serum-free media) or MB231-LEC-CM was added to the bottom chambers. The equilibrated plate was removed from the incubator and 100 μl of the trypsinized cells (45,000 HUVECs per well) with or without inhibitors were added to the top chamber. After 30 min incubation at room temperature (RT), the stabilized chamber was loaded in the RTCA machine and the cell index was measured continuously for 20 h. Cell indices at 20 h were selected for analysis. ACEA E-plates (Roche Diagnostics) were used to measure the extent of HUVEC adhesion. Briefly, HUVECs (25,000 cells per well) in 100 μl of EGM-2 (complete media for HUVECs) or EBM (serum-free media) or MB231-LEC-CM were added. After equilibrating at RT for 30 min, the E-plate was loaded into the RTCA personal system. Cell indices at 3 h were analysed. Cell proliferation assays HUVEC proliferation assays were performed using the WST-1 reagent (Roche) [54] in HUVEC/LEC-CM, EGM or TCM. Two thousand cells per well were plated in 96-well plates and allowed to adhere overnight. On the following day, the media were exchanged with HUVEC/LEC-CM, EGM or TCM. Three days later, the media were replaced with SFM (EBM-2) containing WST-1 reagent and the plates were incubated for 4 h. Changes in colour due to the formazan dye resulting from the cleavage of the tetrazolium salt WST-1 by the mitochondrial succinate-tetrazolium reductase were read on a Victor V fluorescence plate reader (Perkin Elmer, MA) by measuring the absorbance at 450 nm. Tube-formation assays HUVEC/LEC tube-formation assays were performed [54] . Matrigel (50 μl; growth factor reduced, BD Biosciences), thawed on ice at 4 °C overnight, was loaded into each well of a pre-cooled 96-well plate, and the plate was incubated at 37 °C for 30 min. Fifteen thousand HUVECs and LECs in 100 μl LEC-CM were added on top of the matrix in the 96-well plate. For controls, LECs and HUVECs in EC growth media or SFM were also loaded. The plate was then incubated at 37 °C, and the wells were imaged using a Nikon microscope at 20 h (Nikon). TCM-induced metastasis models Animal protocols described in this study were approved by the Institutional Care and Use Committee at the Johns Hopkins Medical Institutions. Before tumour inoculation, we pretreated athymic nude mice (female, 5 weeks, NCI) by injecting 50 μl TCM or GF-dep-TCM or GF/IL6-dep-TCM, or SFM subcutaneously for 2 weeks daily as described previously [7] . After 2 weeks of induction, luc-MB231 cells (2 × 10 6 per mouse, 100 μl of 50% matrigel solution) were injected into the upper inguinal mammary fat pad of the animals under anaesthesia (50 mg kg −1 ketamine and 5 mg kg −1 acepromazine). The tumour size was measured by using a caliper, and the volume was calculated using the formula: V =0.52 × (length) × (width) 2 . We imaged animals every week to track anterior tumour metastases, using the IVIS Xenogen 200 optical imager (Xenogen) after i.p. injection of D-luciferin (Caliper, 150 mg kg −1 ). After 5 weeks, organs were collected and bathed in D-luciferin solution for 5–10 min and placed in the IVIS imager to detect metastases ex vivo . Luciferase-mediated photon flux was quantified by using Living Image 3D Analysis (Xenogen). Maraviroc (8 mg kg −1 , R&D systems) was administered orally daily; anti-hVEGF 165 or anti-mVEGF 164 (5 mg kg −1 , R&D systems) was administered i.p. every 4 days; and S3I-201 (5 mg kg −1 , Calbiochem) was administered intravenously every 2 days. One hundred microlitres of blood was collected from the tail vein, and EDTA plasma was prepared to perform ELISAs. Spontaneous metastasis models without TCM treatment We established MB231 xenograft models as described above without TCM pretreatment. We initiated systemic administration of a CCR5 inhibitor immediately after tumour cell inoculation. The tumour size was measured as described above. We imaged animals every week to track anterior tumour metastases up to 7 weeks, using the IVIS Xenogen 200 optical imager (Xenogen) after i.p. injection of D -luciferin (Caliper, 150 mg kg −1 ). After 7 weeks, organs were collected and bathed in D-luciferin solution for 5–10 min and placed in the IVIS imager to detect metastases ex vivo . LEC-included matrigel plug assays High-concentrated matrigel (500 μl, BD Biosciences) containing LECs or HUVECs (2 × 10 6 per gel) and heparin (10 U per gel) was injected subcutaneously on the ventral side of both flanks of a nude mouse. TCM or SFM (50 μl per injection) were subcutaneously administered daily for 10 days, the mice were killed and the gel plugs were excised and analysed. For visualizing BVs, FITC-dextran (70 kDa, 80 mg kg −1 , Santa Cruz) was injected through the tail vein 1 h before killing. Duration of TCM effect in vivo We assessed time-dependent changes in the concentrations of CCL5 in plasma to understand the duration of the TCM effect in vivo . We treated mice for 2 weeks with TCM or SFM. From week 0 (before the TCM induction), we collected mouse blood samples using the retro-orbital bleeding method, every week up to 7 weeks (four animals per group). We centrifuged the collected blood samples for 20 min at 2,000 g within 30 min of collection, after which the supernatant (EDTA plasma sample) was obtained and stored at −20 °C avoiding repeated freeze–thaw cycles. The samples were analysed using mCCL5 or mVEGF ELISAs. Immunofluorescence Tumours, matrigel plugs, LNs and lungs fixed in 3.5% formalin were placed in 30% sucrose (Sigma) in PBS, incubated overnight at 4 °C and frozen in the optimum cutting temperature (OCT) compound (Sakura). Sections of 10-μm thickness were cut at −20 °C. After blocking with 5% normal goat or normal chicken serum (Jackson Immunoresearch) in phosphate buffered saline Triton (PBST) (0.3% Triton) for 1 h at RT, the sections were treated with one or more of the following primary antibodies overnight at 4 °C: rabbit anti-mouse LYVE-1 antibody (1:200, AngioBio), rat anti-mouse CCL5 (1:200, Abcam), rat anti-mouse CD31 (1:100, BD Pharmingen), goat anti-mouse VEGF 164 , mouse anti-human VEGF 165 (1:300, R&D systems), rabbit anti-pVEGFR2 (1:400, Cell Signaling), mouse anti-smooth muscle actin Cy-3 (1:500, Sigma), rabbit anti-mouse F4/80 (1:100, AbD Serotec), goat anti-mouse lectin FITC (1:100, Sigma), rabbit anti-mouse CD33 antibody (1:50, Santa Cruz), rabbit anti-mouse Iba1 antibody (1:100, Santa Cruz) and rat anti-mouse CD45 (1:200, AbD Serotec). After three rinses with PBST, sections were incubated for 1 h at RT with one or more of the following secondary antibodies (1:500): FITC-conjugated goat anti-rat, FITC-conjugated chicken anti-goat, rhodamine-conjugated goat anti-rat, Cy-3-conjugated goat anti-rabbit, Alexa Fluor 647 goat anti-rabbit, Alexa Fluor 488 goat anti-rabbit, DyLight405 goat anti-rabbit and DyLight405 goat anti-mouse antibodies (all from Jackson Immunoresearch). After three rinses with PBST, the samples were counterstained with 4,6-diamidino-2-phenylindole (DAPI; 1:10,000, Roche; 5 min at RT). The samples were washed with PBST once and mounted with the ProLong Gold anti-fade reagent (Invitrogen) in the dark. Fluorescent signals were visualized and digital images were obtained using the LSM-510 confocal microscope (Carl Zeiss). Histology LNs and lungs were fixed, frozen and sectioned as above. After blocking with 5% goat serum in PBST for 1 h, at RT, the sections were treated with mouse anti-cytokeratin antibodies (1:500, Sigma) overnight at 4 °C. The rest of the 3,3′ diaminobenzidine procedure was performed according to regular protocols [7] . Chromatin immunoprecipitation ChIP was carried out using the EZChip kit (Millipore) according to the manufacturer’s protocol. Five million LECs were seeded into 15 cm plates and grown to 90% confluency in EGM-2MV media. Then, they were treated with 10 ng ml −1 IL6 or vehicle overnight. The cells were cross-linked with 1% formaldehyde for 10 min and sonicated with a Covaris S220 (20% duty cycle, 5 intensity, 200 burst per cycle, 30 cycles of 30 s) for 30 min on ice. The immunoprecipitations were performed using anti-pATF-2, anti-pc-Jun and anti-pStat3 antibodies (all from Cell Signaling) or control IgG and the ChIP DNA in the complex was amplified using the primers for the CCL5 promoter regions. Three regions of the CCL5 promoter with the CRE site (−316 to −69 bp, site 2) and two distal sites (−1,064 to −815 bp, site 1; and −474 to −711 bp, site 3) were tested. The primer sequences for site 1, site 2 and site 3 are 5′-GGGTTCTGATCCCAACTCTG-3′ (forward)/5′-AGCGCGTGTCAACTCATTTA-3′ (reverse); 5′-ACTGCCACTCCTTGTTGTCC-3′ (forward)/5′-GCATTGGCCGGTATCATAAG-3′ (reverse); and 5′-TCTGACTCATGCCTGTCAGC-3′ (forward)/5′-GTGCCAAAATCAGCACAATG-3′ (reverse), respectively. PCR products were analysed by agarose gel electrophoresis and by real-time quantitative PCR. Electrophoretic mobility shift assays The two strands of the wild-type CRE oligonucleotide (5′-AAAGAGGAAACTGATGAGCTCACTCTAGAT-3′) and of mutated CRE (5′-AAAGAGGAAACTGATACAGCCACTCTAGAT-3′), conjugated with biotin at the 5′ end, were synthesized (Invitrogen). Equal amounts of both strands in 0.5 M NaCl, 10 mM Tris, pH 7.5, were annealed by boiling for 5 min at 95 °C, and very gradually cooled on a hot plate. A DNA retardation gel (6%, Novex) was pre-run at 120 V for 50 min at 4 °C. For the binding reaction, 3 μg nuclear extract and 0.5 μg poly(dI-dC) with or without excess unlabelled CRE oligonucleotide were incubated in binding buffer (10 mM Tris, 1 mM EDTA, 50 mM KCl, 10 mM MgCl 2 , 5 μg ml −1 bovine serum albumin, 0.1 mM dithiothreitol) for 10 min at RT, after which oligonucleotide-biotin was added (finally 40 pM) and incubated for 30 min at RT. Ten microlitres of binding sample was mixed with 1 μl 5 × TBE sample buffer (Invitrogen), loaded on the gel and run for 1 h at 120 V in 0.5 × TBE running buffer. The gel was transferred to a DNA transfer stack (Invitrogen), using the iBlot transfer module (Program 8, 7 min). The nylon membrane was dried and cross-linked under a ultraviolet source (305 nm) for 15 min, then probed by the Chemiluminescent Nucleic Acid Detection Module (Pierce). Immunoblot assays For reverse western blot, Proteome Profiler Antibody Array Kits for human angiogenesis factors, chemokines, cytokines and phospho-kinases (R&D systems) were used, according to the manufacturer’s instructions. For western blot, 400,000 MDA-MB-231 or LECs (per well) were starved for 24 h, after which they were treated with Stattic (5–10 μM), S3I-201 (2.5–10 μM) or SP600125 (40 μM) and incubated for 60 min. After that, inducers, including TCM (30%), EGM, IL6-dep-TCM, IL6 or EGF, were added. We followed the standard protocol for the rest of the procedure as described previously [11] applying antibodies of interest, including pStat3, HIF-1α, gp130, pNFkB, NFkB, IkBα, Stat3, pCREB, GAPDH (glyceraldehyde 3-phosphate dehydrogenase; all from Cell Signaling), pc-Jun, pATF-2 (Sigma), CCR5 and Lamin B1 (Abcam). All the original gel images of immunoblot analyses are presented in Supplementary Fig. 25 . Co-immunoprecipitation LECs (2 × 10 6 ) treated with Stattic, SP600125, IL6 or EGM were used to prepare cell lysates or nuclear extracts. Five hundred microlitres of cell lysates or 200 μl nuclear extracts were incubated overnight at 4 °C with antibodies suitable for IP (1:100 diluted): pStat3, pc-Jun, pATF-2, pNFkB and NFkB (Cell Signaling). Ten microlitres of Protein A/G Plus Agarose (Santa Cruz Biotech) was added and incubated for 3 h at 4 °C. The beads were rinsed three times with 500 μl cell lysis buffer for IP (Pierce) supplemented with the protease inhibitor and phosphatase inhibitor cocktail 2/3 (Sigma). The protein complex was reduced and separated by SDS–polyacrylamide gel electrophoresis and probed with the following antibodies in a western assay: pStat3, pc-Jun, pATF-2, pNFkB and NFkB (Sigma). All the original gel images of immunoblot analyses are presented in Supplementary Fig. 25 . Lung vascular permeability assays After 2 weeks of TCM or SFM treatment with or without anti-VEGF antibodies, FITC-dextran was injected intravenous through the tail vein (70 kDa, 80 mg kg −1 ) 1 h before killing. Collected lungs were stained with mCD31 and observed under the LSM-510 confocal microscope. HUVEC monolayer integrity assays HUVECs (10,000 cells) in complete media (200 μl) were plated in fibronectin-coated eight-well Lab Tek chamber slides (Cole Palmer). After starving cells in 2% FBS-based serum-free media (no bullet kit) overnight, TCM or GF-dep-TCM or LEC-CM with or without anti-hVEGF 165 (50 μg ml −1 , R&D systems) were added for 4 h. The cells were fixed for 10 min in 3.5% formalin in PBS, and incubated for 5 min on ice in 0.5% Triton X-100 in PBS. After blocking with 2% bovine serum albumin or 5% normal goat serum, the monolayers were processed for staining with anti-ZO-1 FITC (1:500, Cell Signaling), anti-phalloidin rhodamine (1:500, Molecular probe), rabbit anti-cleaved caspase 3 (1:500, Cell Signaling) and DAPI (1:10,000, Roche). Fluorescence images were obtained using a LSM-510 confocal microscope (Carl Zeiss). TCGA data analyses All analyses of TCGA primary breast cancer tissues [55] were performed in R (3.0.1). TCGA Level 3, RSEM v2 gene expression measurements from RNA sequencing for CCL5 and IL6 were obtained from the cBioPortal with the CRAN cgdsr package [56] . ER and PR status were obtained from cross-platform summaries, and HER2 status from IHC measurements in the TCGA clinical data, with a total of 99 triple-negative samples and 326 ER+/PR+/HER2−. Samples were called LN positive if at least one LN was positive by either IHC or hematoxylin and eosin staining, consistent with pathological staging in the TCGA clinical annotations ( Supplementary Methods ). There were 50 LN-negative and 37 LN-positive samples within the TNBC subtype. We compared expression between subtypes with one-sided t -tests on log-transformed RSEM values. Correlation coefficients and corresponding P values were computed with Pearson’s correlation. All the codes are described in the Supplementary Methods . Statistical analysis Error bars correspond to s.e.m., unless otherwise stated. Differences between two groups are regarded as significant when P is <0.05 using the Student’s t -test. How to cite this article: Lee, E. et al. Breast cancer cells condition lymphatic endothelial cells within pre-metastatic niches to promote metastasis. Nat. Commun. 5:4715 doi: 10.1038/ncomms5715 (2014).